Arf6 regulates tumour angiogenesis and growth through HGF-induced endothelial β1 integrin recycling Anti-angiogenic drugs targeting vascular endothelial cell growth factor receptor have provided modest clinical benefit, in part, owing to the actions of additional angiogenic factors that stimulate tumour neoangiogenesis in parallel. To overcome this redundancy, approaches targeting these other signalling pathways are required. Here we show, using endothelial cell-targeted mice, that the small GTPase Arf6 is required for hepatocyte growth factor (HGF)-induced tumour neoangiogenesis and growth. Arf6 deletion from endothelial cells abolishes HGF-stimulated β1 integrin recycling. Pharmacological inhibition of the Arf6 guanine nucleotide exchange factor (GEF) Grp1 efficiently suppresses tumour vascularization and growth. Grp1 as well as other Arf6 GEFs, such as GEP100, EFA6B and EFA6D, regulates HGF-stimulated β1 integrin recycling. These findings provide insight into the mechanism of HGF-induced tumour angiogenesis and offer the possibility that targeting the HGF-activated Arf6 signalling pathway may synergize with existing anti-angiogenic drugs to improve clinical outcomes. Tumour-associated angiogenesis is one of the hallmarks underlying cancer development [1] . Neovascularization in tumours supplies oxygen and nutrients, thereby being essential for the tumour growth beyond a relatively small size; inhibition of neoangiogenesis leads to tumour stasis [2] , [3] . Among angiogenic growth factors secreted from tumour cells or tumour stroma cells, vascular endothelial cell growth factor (VEGF) is one of the most important factor [4] . During the past decade, anti-angiogenic drugs targeting VEGF receptor (VEGFR) signalling such as bevacizumab, a humanized VEGF-neutralizing monoclonal antibody, and sunitinib, a tyrosine kinase inhibitor that targets VEGFR, and the platelet-derived growth factor (PDGF) receptor (PDGFR), have been developed [3] . However, the clinical benefits obtained using them have been relatively modest [5] . It has been proposed that tumours adapt and reinitiate growth via a process referred to as angiogenic redundancy in which compensatory angiogenic growth factors are produced to overcome VEGFR signalling inhibition [5] , [6] . Hence, the evasion mechanisms evoked by targeting a single pathway represents a major therapeutic obstacle. The hepatocyte growth factor (HGF)/cMet axis is a potent mitogenic, motogenic and morphogenic pathway [7] , [8] that can drive tumour angiogenesis and growth [9] , [10] , [11] . Expression of cMet and HGF is observed in the vast majority of solid tumours [12] . Activation of cMet stimulates proliferation, survival and invasiveness of cancer cells through several signalling pathways mediated by phosphatidylinositol 3-kinase/Akt, Src, STAT3 and Ras/mitogen-activated protein kinase (MAPK) [8] . In the vasculature, cMet activation through paracrine signalling by tumour cell-released HGF stimulates tumour angiogenesis by inducing proliferation, migration and survival of endothelial cells [13] . Expression of both cMet and HGF is induced by hypoxia-inducible factor 1α, further providing evidence for an important role of the HGF/cMet axis in adverse microenvironment conditions to promote tumour angiogenesis [14] , [15] . Importantly, it has been reported in a preclinical model that HGF/cMet signalling can act as an alternative angiogenic pathway in sunitinib-resistant tumours [16] . These observations indicate that targeting HGF/cMet signalling pathway in endothelial cells might be an effective approach to overcome the evasive resistance of cancer cells in the context of angiogenesis redundancy. However, the molecular mechanisms underlying how the HGF/cMet axis regulates tumour angiogenesis are poorly understood. The small GTPase Arf6 plays important roles in cell migration and membrane dynamics by regulating intracellular membrane trafficking and reorganizing the actin cytoskeleton [17] , [18] . Arf6 cycles through a GDP-bound inactive and a GTP-bound active form. Guanine nucleotide exchange factors (GEFs) facilitate the exchange of GDP for GTP to generate the Arf6 active form that then binds to and regulates downstream effectors [19] . We and others have reported that Arf6 is involved in HGF-induced signalling pathways [20] , [21] . Genetic ablation of Arf6 in mice induces abnormal fetal liver development, resulting in embryonic lethality in mid-gestation [22] . In an in vitro system, hepatocytes isolated from Arf6 knockout (KO; Arf6 −/− ) embryos exhibit impaired morphological responses to HGF stimulation and defective hepatic cord formation [22] . These observations led us to speculate that Arf6 might be involved in HGF-stimulated tumour angiogenesis. In support of this proposal, Arf6 has recently been shown to be involved in angiogenesis-related cell functions in vitro [23] , [24] , [25] , [26] . However, the in vivo functions of Arf6 in endothelial cells, in particular in relationship to HGF-regulated tumour angiogenesis and growth, have not been explored. Here, we show that Arf6 exerts a role required in endothelial cells to support HGF-induced tumour angiogenesis and growth. In endothelial cells, Arf6 is essential for HGF, but not VEGF-dependent β1 integrin recycling to the plasma membrane, and promotes endothelial cell adhesion and migration. The Arf6 GEF, Grp1, localizes at the β1 integrin-positive intracellular compartment, and is involved in HGF-dependent Arf6 activation, β1 integrin recycling and tumour angiogenesis and growth in mice. These findings define the molecular mechanisms underlying HGF-induced tumour angiogenesis, and provide us new therapeutic opportunities to control angiogenesis in tumour. Endothelial Arf6 regulates tumour angiogenesis and growth In situ hybridization of Arf6 messenger RNA (mRNA) expression in E13.5 mouse embryos revealed transcripts in neural tube blood vessels ( Fig. 1a ) and in vascular endothelial, smooth muscle and mesenchymal cells surrounding the dorsal aorta, with the highest levels of expression in the vascular endothelial cells ( Fig. 1b ), suggesting a potential role for Arf6 in angiogenesis. To explore this hypothesis, conditional KO mice in which Arf6 gene was deleted from endothelial cells (EC- Arf6 cKO) were generated ( Fig. 1c–e and Supplementary Fig. 1a,b ) by mating Arf6 flox/flox mice with Tie2-Cre mice [27] . EC- Arf6 cKO mice were born at the expected Mendelian ratio, and were overtly healthy and fertile ( Supplementary Fig. 1c,d ). Angiogenesis in the head and neck of EC- Arf6 cKO embryonic mice and in the P5 neonatal retina was similar to that of control Arf6 flox/flox mice, although the vascular length in the dorsal torso was slightly decreased ( Supplementary Figs 2 and 3 ). Nonetheless, these findings indicated that endothelial Arf6 is not crucial for embryogenesis. 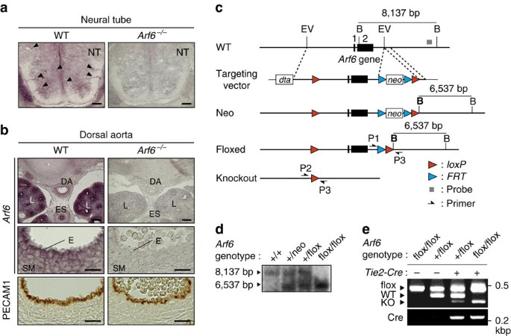Figure 1: Expression ofArf6mRNA in blood vessels and conditional targeting of endothelial Arf6. (a)In situhybridization forArf6mRNA of neural tube blood vessels. Arrow heads in the left panel indicate vessels sprouting into the neural tube of the wild-type (WT) embryo. (b)In situhybridization forArf6(top and middle panels) and immunostaining for PECAM1 (bottom panels) in dorsal aorta of E13.5 embryos. High-magnification images of the rim of aortas (middle panels) showArf6expression in the endothelium of WT embryo. NT, neural tube; SM, smooth muscle layer; E, endothelium; ES, oesophagus; DA, dorsal aorta; L, lung. Scale bar, 100 μm. (c) Schematic representation of the conditional gene targeting strategy forArf6. Exons forArf6are represented by filled black rectangles. The neomycin-resistance selection cassette is represented as ‘neo’.loxPandFRTsites, red and blue triangles, respectively. EV, B; restriction sites for EcoRV and BamHI. Targeting vector-derived restriction sites are shown in bold. The relevant restriction fragments for Southern blotting are shown by horizontal lines with fragment sizes. A probe fragment for Southern blotting is represented by a grey box. Positions of primers used for genomic PCR analysis are shown by arrows. (d) Southern blot analysis of BamHI-digested genomic DNAs from each genotype of mouse tails using probe indicated inc. (e) Genomic PCR analysis of the offspring of aTie2-Cre;Arf6flox/+male andArf6flox/floxfemale pair. DNA fragments amplified from KO, WT and floxed alleles (flox) were detected. Figure 1: Expression of Arf6 mRNA in blood vessels and conditional targeting of endothelial Arf6. ( a ) In situ hybridization for Arf6 mRNA of neural tube blood vessels. Arrow heads in the left panel indicate vessels sprouting into the neural tube of the wild-type (WT) embryo. ( b ) In situ hybridization for Arf6 (top and middle panels) and immunostaining for PECAM1 (bottom panels) in dorsal aorta of E13.5 embryos. High-magnification images of the rim of aortas (middle panels) show Arf6 expression in the endothelium of WT embryo. NT, neural tube; SM, smooth muscle layer; E, endothelium; ES, oesophagus; DA, dorsal aorta; L, lung. Scale bar, 100 μm. ( c ) Schematic representation of the conditional gene targeting strategy for Arf6 . Exons for Arf6 are represented by filled black rectangles. The neomycin-resistance selection cassette is represented as ‘ neo’ . loxP and FRT sites, red and blue triangles, respectively. EV, B; restriction sites for EcoRV and BamHI. Targeting vector-derived restriction sites are shown in bold. The relevant restriction fragments for Southern blotting are shown by horizontal lines with fragment sizes. A probe fragment for Southern blotting is represented by a grey box. Positions of primers used for genomic PCR analysis are shown by arrows. ( d ) Southern blot analysis of BamHI-digested genomic DNAs from each genotype of mouse tails using probe indicated in c . ( e ) Genomic PCR analysis of the offspring of a Tie2-Cre;Arf6 flox/+ male and Arf6 flox/flox female pair. DNA fragments amplified from KO, WT and floxed alleles (flox) were detected. Full size image Interestingly, growth of B16 melanoma and Lewis lung carcinoma (LLC) tumours subcutaneously transplanted into the EC- Arf6 cKO mice were significantly reduced in comparison with tumours implanted into control Arf6 flox/flox mice ( Fig. 2a,b ). Concomitantly, tumour angiogenesis was impaired in the EC- Arf6 cKO mice as assessed by vascular area and blood vessel number in the syngrafts ( Fig. 2c,d ), with fewer numbers of α-SMA + vessels and mature vessels with open lumens ( Fig. 1e,f and Supplementary Fig. 4 ). These results suggest that Arf6 in endothelial cells plays a crucial role in tumour angiogenesis, thereby regulating tumour growth. Since Tie2 is expressed in haematopoietic as well as endothelial cells [28] and Tie2-expressing bone marrow-derived monocytes have been reported to promote tumour angiogenesis in mouse tumour models [29] , [30] , we examined the possibility that ablation of Arf6 in haematopoietic cells contributed to or created the tumour angiogenesis phenotype by performing bone marrow transplantations. Bone marrow reconstitution efficiency was assessed by determining the frequency of Ly5.1 + haematopoietic cells in the Ly5.2-expressing recipient mice ( Supplementary Fig. 5a ). B16 and LLC tumour growth and angiogenesis continued to be suppressed in EC- Arf6 cKO mice reconstituted with control bone marrow cells, and tumour growth and angiogenesis in control mice was not suppressed by reconstitution with bone marrow cells prepared from EC- Arf6 cKO mice ( Supplementary Fig. 5b–d ), demonstrating that Arf6 expressed in endothelial cells, but not in bone marrow-derived cells, plays an important role in tumour angiogenesis and growth. 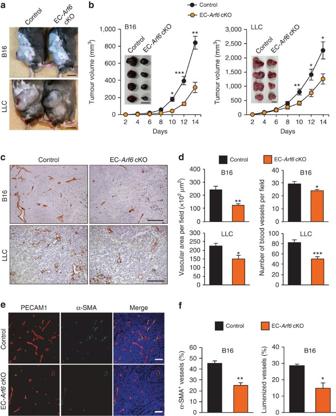Figure 2: Inhibition of tumour growth and angiogenesis in EC-Arf6cKO mice. (a,b) Growth of B16 melanoma and LLC syngraft tumours. Pictures shown inaare primary tumours after 14 days of transplantation.n=8 and *P<0.0005, **P<0.0001, ***P<0.00005 (b, left).n=20 and 18 for control and EC-Arf6cKO, respectively, and *P<0.01, **P<0.005 (b, right). Scale bars, 1 cm. (c–f) Tumour angiogenesis analysed by immunostaining for the marker protein platelet-endothelial cells adhesion molecules 1 (PECAM1) (c,d) and α-SMA (e,f) in sections of B16 or LLC tumours after 14 days of transplantation. Vascular area (d, left), number of vessels (d, right), vessels covered by α-SMA+mural cells (f, left) and percentage of lumenized vessels (f, right) were quantified.n≥5. *P<0.05, **P<0.005 and ***P<0.001 (d), and *P<0.005 and **P<0.0005 (f). Scale bars, 200 μm (c) and 100 μm (e). Means±s.e.m. were shown for all panels. Statistical analyses were performed using Student’st-test. Figure 2: Inhibition of tumour growth and angiogenesis in EC- Arf6 cKO mice. ( a , b ) Growth of B16 melanoma and LLC syngraft tumours. Pictures shown in a are primary tumours after 14 days of transplantation. n =8 and * P <0.0005, ** P <0.0001, *** P <0.00005 ( b , left). n =20 and 18 for control and EC- Arf6 cKO, respectively, and * P <0.01, ** P <0.005 ( b , right). Scale bars, 1 cm. ( c – f ) Tumour angiogenesis analysed by immunostaining for the marker protein platelet-endothelial cells adhesion molecules 1 (PECAM1) ( c , d ) and α-SMA ( e , f ) in sections of B16 or LLC tumours after 14 days of transplantation. Vascular area ( d , left), number of vessels ( d , right), vessels covered by α-SMA + mural cells ( f , left) and percentage of lumenized vessels ( f , right) were quantified. n ≥5. * P <0.05, ** P <0.005 and *** P <0.001 ( d ), and * P <0.005 and ** P <0.0005 ( f ). Scale bars, 200 μm ( c ) and 100 μm ( e ). Means±s.e.m. were shown for all panels. Statistical analyses were performed using Student’s t -test. Full size image Arf6 regulates HGF-induced angiogenesis To investigate which angiogenic growth factor links to the Arf6-dependent signalling pathway regulating tumour angiogenesis, we used the Arf6 flox/flox mice to generate immortalized endothelial cells (iECs) as defined by being PECAM1 -, ICAM2 - and endomucin positive, and NG2 - and PDGFRβ negative ( Supplementary Fig. 6a ). Infection of recombinant adenoviruses expressing Cre recombinase into the Arf6 flox/flox iECs ablated Arf6 with high efficiency, whereas infection of control virus encoding LacZ was without effect on the expression level of Arf6 protein ( Supplementary Fig. 6b,c ). Stimulation of the iECs with recombinant VEGF-A 165 (VEGF), basic fibroblast growth factor (bFGF) and HGF triggered capillary tube formation ( Fig. 3a,b ). Whereas the VEGF- and bFGF-stimulated responses were unaltered in the absence of Arf6, the HGF-induced response was decreased by ∼ 60% in Arf6 −/− iECs (increases in tube lengths of control and Arf6 −/− iECs in response to HGF stimulation were 1.07 (2.67–1.60) and 0.41 (1.98–1.57) mm mm −2 , respectively). Similarly, deletion of Arf6 from endothelial cells markedly inhibited HGF-induced, but not VEGF- or bFGF-induced, microvessel outgrowth from aortic ring explants ( Fig. 3c,d ). These results, taken together with the report linking HGF/cMet signalling in endothelial cells to tumour angiogenesis and growth [9] , [10] , [11] , led us to hypothesize that activation of Arf6 is a critical step in the HGF-dependent signalling pathway coupled to tumour angiogenesis. In support of this hypothesis, Arf6 was activated upon HGF stimulation of endothelial cells ( Fig. 3e ). VEGF stimulation also activated Arf6, but very rapidly and only transiently ( Fig. 3f ), indicating that Arf6 might also play a role(s) in VEGF-dependent cell signalling coupling to a cell function(s) other than in vitro capillary tube formation and aortic microvessel sprouting. In further support, HGF was found to be expressed in B16 and LLC tumour syngrafts at both mRNA and protein levels, although protein levels of HGF in the cancer cells cultured in vitro were below detection ( Supplementary Fig. 7 ), suggesting that expression of HGF by the tumour cells is regulated in vivo in a context-dependent manner such as in the setting of hypoxia or nutrient stress. 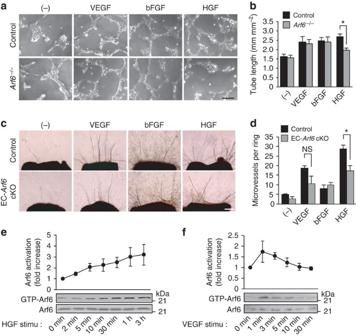Figure 3: HGF-dependentin vitroangiogenesis is mediated by Arf6. (a,b) Angiogenic factor-inducedin vitrocapillary tube formation by control andArf6−/−iECs. Scale bar, 50 μm. (c,d) Angiogenic factor-induced microvessel sprouting from aortic ring explants prepared from control and EC-Arf6cKO mice. Scale bar, 200 μm. (e,f) Time-dependent activation of Arf6 upon HGF (e) and VEGF-A stimulation (stimu) (f). Means±s.e.m. from at least three independent experiments were shown for all panels. *P<0.05; NS, not significant, Student’st-test forband one-way analysis of variance with Tukey’s multiple comparison test ford. Figure 3: HGF-dependent in vitro angiogenesis is mediated by Arf6. ( a , b ) Angiogenic factor-induced in vitro capillary tube formation by control and Arf6 −/− iECs. Scale bar, 50 μm. ( c , d ) Angiogenic factor-induced microvessel sprouting from aortic ring explants prepared from control and EC- Arf6 cKO mice. Scale bar, 200 μm. ( e , f ) Time-dependent activation of Arf6 upon HGF ( e ) and VEGF-A stimulation (stimu) ( f ). Means±s.e.m. from at least three independent experiments were shown for all panels. * P <0.05; NS, not significant, Student’s t -test for b and one-way analysis of variance with Tukey’s multiple comparison test for d . Full size image Arf6 is essential for cell spreading and focal adhesion Angiogenic growth factor-dependent proliferation and migration of endothelial cells are essential events for angiogenesis [3] . Although deletion of Arf6 was without effect on HGF- and fetal bovine serum (FBS)-stimulated proliferation ( Supplementary Fig. 8 ), cell migration toward HGF was almost completely inhibited for Arf6 −/− iECs ( Fig. 4a ). This inhibition is unlikely to be attributable to an abnormality in the HGF receptor cMet: expression and cell surface levels, HGF-stimulated phosphorylation at Y1234/Y1235, degradation, internalization and recycling of cMet in Arf6 −/− iECs were essentially identical to those observed for control iECs ( Supplementary Fig. 9 ). Although it has been reported that Arf6 is required for activation of MAPK ERK1/2 and the small G protein Rac1 in HGF-stimulated epithelial cells [20] , which are implicated in endothelial cell migration [31] , [32] , no difference in activation of MAPKs, such as ERK1/2, p38 and JNK, Akt and Rac1 was observed for Arf6 −/− iECs in comparison with control iECs ( Supplementary Fig. 10 ), eliminating these signalling pathways and outputs from further consideration. 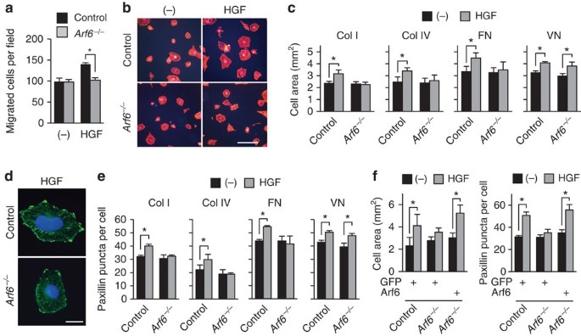Figure 4: Arf6 regulates HGF-induced migration, spreading and FA of endothelial cells. (a) Inhibition of HGF-induced cell migration byArf6deletion from iECs. (b–e) Inhibition of HGF-dependent cell spreading (b,c) and FA (d,e) byArf6deletion from iECs. Control andArf6−/−iECs were cultured on collagen type I (Col I; 0.3 mg ml−1;b–e), collagen type IV (Col IV; 5 μg ml−1), fibronectin (FN; 10 μg ml−1) or vitronectin (VN; 10 μg ml−1;c,e), and stained for F-actin (b) or paxillin (green)/DAPI (blue) (d). Cell area (c) and number of paxillin puncta (e) were measured and represented as described inSupplementary Fig. 11. Scale bars, 100 μm (b) and 20 μm (d). (f) Rescue of HGF-dependent cell spreading (left) and FA (right) by ectopic expression of Arf6 inArf6−/−iECs. Data were shown as means±s.e.m. from three independent experiments in which >150 (c), 100 (e) and 40 cells (f) were assessed. *P<0.05; NS, not significant, one-way analysis of variance with Tukey’s multiple comparison test foraand Student’st-test forc,e,f. Figure 4: Arf6 regulates HGF-induced migration, spreading and FA of endothelial cells. ( a ) Inhibition of HGF-induced cell migration by Arf6 deletion from iECs. ( b – e ) Inhibition of HGF-dependent cell spreading ( b , c ) and FA ( d , e ) by Arf6 deletion from iECs. Control and Arf6 −/− iECs were cultured on collagen type I (Col I; 0.3 mg ml −1 ; b – e ), collagen type IV (Col IV; 5 μg ml −1 ), fibronectin (FN; 10 μg ml −1 ) or vitronectin (VN; 10 μg ml −1 ; c , e ), and stained for F-actin ( b ) or paxillin (green)/DAPI (blue) ( d ). Cell area ( c ) and number of paxillin puncta ( e ) were measured and represented as described in Supplementary Fig. 11 . Scale bars, 100 μm ( b ) and 20 μm ( d ). ( f ) Rescue of HGF-dependent cell spreading (left) and FA (right) by ectopic expression of Arf6 in Arf6 −/− iECs. Data were shown as means±s.e.m. from three independent experiments in which >150 ( c ), 100 ( e ) and 40 cells ( f ) were assessed. * P <0.05; NS, not significant, one-way analysis of variance with Tukey’s multiple comparison test for a and Student’s t -test for c , e , f . Full size image Cell spreading and focal adhesion (FA) formation are both important for cell migration [33] , [34] . HGF-induced cell spreading and FA formation were almost completely inhibited when Arf6 −/− iECs were cultured on the β1 integrin ligands collagen type I, collagen type IV and fibronectin, but not for the β3 integrin ligand vitronectin ( Fig. 4b–e and Supplementary Fig. 11 ). The inhibition was rescued in full by ectopic expression of Arf6 in the Arf6 −/− iECs ( Fig. 4f and Supplementary Fig. 12 ). These results raised the possibility that Arf6 regulates HGF-dependent cell spreading and FA formation in vascular endothelial cells by controlling activation and/or recycling of β1 integrin back to the plasma membrane. Arf6 regulates HGF-induced β1 integrin recycling Arf6 located at endosomes has been proposed to regulate serum-dependent recycling of β1 integrin [35] , [36] . However, HGF signalling has not been studied in this context. Stimulation of iECs with HGF increased β1 integrin surface levels within 5 min ( Fig. 5a ). In contrast, no β1 integrin recycling occurred in response to HGF for Arf6 −/− iECs. Providing specificity for this result, VEGF-stimulated β1 integrin recycling was identical in control and Arf6 −/− iECs ( Fig. 5b ). Consistent with this observation, HGF-dependent recycling of β1 integrin from intracellular compartment(s) to the plasma membrane, as assessed by immunostaining for internal β1 integrin, was significantly suppressed in Arf6 −/− iECs ( Fig. 5c ). Overexpression of β1 integrin in Arf6 −/− iECs could not rescue the defect in HGF-induced in vitro tube formation ( Supplementary Fig. 13 ), indicating that Arf6-regulated β1 recycling to the plasma membrane is critical. The impairment of β1 integrin recycling by Arf6 deletion was not attributable to the inhibition of endocytosis of β1 integrin, since HGF-dependent internalization of β1 integrin at the plasma membrane was induced in Arf6 −/− iECs to the same extent as in control cells ( Fig. 5d ). We also found that the HGF-stimulated level of the active form of β1 integrin at the plasma membrane, which was immunochemically detected using the conformation-sensitive antibody 9EG7 (ref. 37 ), was significantly decreased for Arf6 −/− iECs ( Fig. 5e ), and this was observed as well for tumour vessels lacking Arf6 ( Fig. 5f ). Although this observation can be explained by the inhibition of β1 integrin recycling, we cannot totally exclude the possibility that Arf6 also directly regulates activation of β1 integrin at the plasma membrane. Nonetheless, inhibition of HGF-induced FA formation in Arf6 −/− iECs seems clearly to be attributable to reduced amounts of the active form of β1 integrin at the plasma membrane, thereby causing defective spreading and migration. 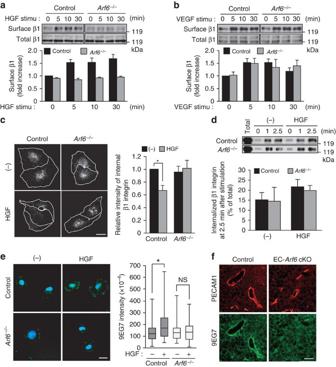Figure 5: Arf6 is required for HGF-induced β1 integrin recycling/activation in endothelial cells. (a,b) Effects ofArf6deletion on surface β1 integrin level in HGF- and VEGF-stimulated iECs. After stimulation of cells with HGF (a) and VEGF (b) for the indicated times, β1 integrin levels at the plasma membrane of control andArf6−/−iECs were detected (upper panels) as described in Methods section. The data were quantified and represented as means±s.e.m. from three independent experiments (lower panels). (c) Effects ofArf6deletion on HGF-induced recycling of β1 integrin from internal compartments to the plasma membrane in iECs. Internal β1 integrin labelled with anti-β1 integrin antibody (HMβ1-1) were detected by immunostaining after stimulation of cells with or without HGF and following wash out of cell surface antibody (c, left), and its fluorescence intensity was measured (c, right). Means±s.e.m. from four independent experiments were shown. Scale bar, 20 μm. (d) Effects ofArf6deletion on HGF-induced internalization of β1 integrin by iECs. Biotin-labelled surface β1 integrin were internalized by incubating with or without HGF and internal β1 integrin were detected as described in Methods section. Means±s.e.m. from three independent experiments were shown. (e) Inhibition of HGF-induced β1 integrin recycling/activation byArf6deletion from iECs. The active form of β1 integrin was immunostained with the antibody 9EG7 (green;e, left), and its intensity from three independent experiments was measured for >50 cells (e, right; median, quartiles, maximum and minimum values are indicated). Cells were also stained with DAPI (blue). Scale bar, 20 μm. (f) Immunostaining for active form of β1 integrin in blood vessels of B16 melanoma tumours produced in control and EC-Arf6cKO mice. Scale bar, 50 μm. *P<0.05; NS, not significant, Student’st-test forcand non-parametric Mann–WhitneyU-test fore. Figure 5: Arf6 is required for HGF-induced β1 integrin recycling/activation in endothelial cells. ( a , b ) Effects of Arf6 deletion on surface β1 integrin level in HGF- and VEGF-stimulated iECs. After stimulation of cells with HGF ( a ) and VEGF ( b ) for the indicated times, β1 integrin levels at the plasma membrane of control and Arf6 −/− iECs were detected (upper panels) as described in Methods section. The data were quantified and represented as means±s.e.m. from three independent experiments (lower panels). ( c ) Effects of Arf6 deletion on HGF-induced recycling of β1 integrin from internal compartments to the plasma membrane in iECs. Internal β1 integrin labelled with anti-β1 integrin antibody (HMβ1-1) were detected by immunostaining after stimulation of cells with or without HGF and following wash out of cell surface antibody ( c , left), and its fluorescence intensity was measured ( c , right). Means±s.e.m. from four independent experiments were shown. Scale bar, 20 μm. ( d ) Effects of Arf6 deletion on HGF-induced internalization of β1 integrin by iECs. Biotin-labelled surface β1 integrin were internalized by incubating with or without HGF and internal β1 integrin were detected as described in Methods section. Means±s.e.m. from three independent experiments were shown. ( e ) Inhibition of HGF-induced β1 integrin recycling/activation by Arf6 deletion from iECs. The active form of β1 integrin was immunostained with the antibody 9EG7 (green; e , left), and its intensity from three independent experiments was measured for >50 cells ( e , right; median, quartiles, maximum and minimum values are indicated). Cells were also stained with DAPI (blue). Scale bar, 20 μm. ( f ) Immunostaining for active form of β1 integrin in blood vessels of B16 melanoma tumours produced in control and EC- Arf6 cKO mice. Scale bar, 50 μm. * P <0.05; NS, not significant, Student’s t -test for c and non-parametric Mann–Whitney U -test for e . Full size image β1 Integrin recycling is dependent on Arf6 GEFs Seven of the 11 Arf GEFs thus far identified, BRAG2/GEP100, EFA6A-D, cytohesin2/ARNO and cytohesin3/Grp1, function as Arf6 GEFs [19] . mRNAs for all of the Arf6 GEFs were found to be expressed in both iECs and human umbilical vascular endothelial cells (HUVECs; Supplementary Fig. 14a ), the latter of which is widely used as a model cell for physiological studies of endothelial cells. To examine whether the cytohesins function upstream of Arf6 in the HGF/cMet-dependent β1 integrin recycling signalling pathway, SecinH3, a cytohesin family-specific inhibitor [38] , was used. SecinH3 significantly inhibited HGF-dependent Arf6 activation and the increase of surface β1 integrin level in control iECs ( Fig. 6a,b ). 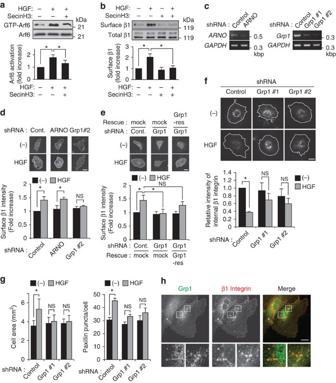Figure 6: Grp1 is essential for β1 integrin recycling. (a) Inhibition of HGF-induced Arf6 activation by SecinH3 in iECs. After HGF stimulation of cells pretreated with SecinH3, the GTP-bound Arf6 was detected. (b) Inhibition of HGF-induced β1 integrin recycling by SecinH3 in iECs. β1 Integrin on the plasma membrane was detected as inFig. 5a. (c) Efficacy of shRNAs for ARNO and Grp1 in HUVECs as assessed by RT–PCR. (d) Effects of cytohesin knockdown on HGF-dependent β1 integrin translocation to the plasma membrane in HUVECs. Cell surface β1 integrin was immunostained after stimulation with or without HGF. The fluorescence intensities at the plasma membrane were measured for >18 cells in each experiment. Scale bar, 40 μm. (e) Rescue of HGF-dependent β1 integrin translocation to the plasma membrane by ectopic expression of shRNA-resistant Grp1 (Grp1-res). GFP (mock) or GFP-Grp1-res was expressed in Grp1-knocked-down HUVECs (shRNA # 2 for Grp1), and cell surface β1 integrin was immunostained after stimulation with or without HGF. The fluorescence intensity of surface β1 integrin was measured for >25 cells in the lower panel. Scale bar, 40 μm. (f) Inhibition of HGF-dependent β1 integrin recycling by Grp1 knockdown in HUVECs. Internal β1 integrin after stimulation with or without HGF was immunostained with anti-β1 integrin antibody (TS2/16). The internal β1 integrin intensity was measured for >20 cells in the lower panel. Scale bar, 20 μm. (g) Inhibition of HGF-induced spreading (left panel) and FA formation (right panel) by Grp1 knockdown. HUVECs cultured on collagen type I were measured for cell area and number of paxillin puncta. (h) Co-localization of endogenous Grp1 and β1 integrin at the intracellular compartments. Grp1 (green) and β1 integrin (red) in HUVECs cultured with HGF on collagen type I were detected. Scale bar, 20 μm. Quantitative data are shown as means±s.e.m from more than three independent experiments. *P<0.05; NS, not significant, one-way analysis of variance with Dunnett’s multiple comparison test for (a,b,e) and Student’st-test for (d,f,g). Figure 6: Grp1 is essential for β1 integrin recycling. ( a ) Inhibition of HGF-induced Arf6 activation by SecinH3 in iECs. After HGF stimulation of cells pretreated with SecinH3, the GTP-bound Arf6 was detected. ( b ) Inhibition of HGF-induced β1 integrin recycling by SecinH3 in iECs. β1 Integrin on the plasma membrane was detected as in Fig. 5a . ( c ) Efficacy of shRNAs for ARNO and Grp1 in HUVECs as assessed by RT–PCR. ( d ) Effects of cytohesin knockdown on HGF-dependent β1 integrin translocation to the plasma membrane in HUVECs. Cell surface β1 integrin was immunostained after stimulation with or without HGF. The fluorescence intensities at the plasma membrane were measured for >18 cells in each experiment. Scale bar, 40 μm. ( e ) Rescue of HGF-dependent β1 integrin translocation to the plasma membrane by ectopic expression of shRNA-resistant Grp1 (Grp1-res). GFP (mock) or GFP-Grp1-res was expressed in Grp1-knocked-down HUVECs (shRNA # 2 for Grp1), and cell surface β1 integrin was immunostained after stimulation with or without HGF. The fluorescence intensity of surface β1 integrin was measured for >25 cells in the lower panel. Scale bar, 40 μm. ( f ) Inhibition of HGF-dependent β1 integrin recycling by Grp1 knockdown in HUVECs. Internal β1 integrin after stimulation with or without HGF was immunostained with anti-β1 integrin antibody (TS2/16). The internal β1 integrin intensity was measured for >20 cells in the lower panel. Scale bar, 20 μm. ( g ) Inhibition of HGF-induced spreading (left panel) and FA formation (right panel) by Grp1 knockdown. HUVECs cultured on collagen type I were measured for cell area and number of paxillin puncta. ( h ) Co-localization of endogenous Grp1 and β1 integrin at the intracellular compartments. Grp1 (green) and β1 integrin (red) in HUVECs cultured with HGF on collagen type I were detected. Scale bar, 20 μm. Quantitative data are shown as means±s.e.m from more than three independent experiments. * P <0.05; NS, not significant, one-way analysis of variance with Dunnett’s multiple comparison test for ( a , b , e ) and Student’s t -test for ( d , f , g ). Full size image The cytohesin family is composed of four members [19] . Since activity of cytohesin1 and cytohesin4 for Arf6 has not yet been established, we focused on cytohesin2 (also known as ARNO) and cytohesin3 (also known as Grp1). Knockdown of Grp1, but not ARNO, in HUVECs by short hairpin RNAs (shRNAs; Fig. 6c ) almost completely inhibited HGF-dependent increases in β1 integrin at the plasma membrane ( Fig. 6d ): HGF-stimulated surface β1 integrin levels in the Grp1-knocked-down cells was almost the same as unstimulated levels as assessed by immunostaining of cell surface β1 integrin. The inhibition of β1 integrin recycling by Grp1 knockdown was rescued by the ectopic expression of shRNA-resistant Grp1 ( Fig. 6e ). Furthermore, the HGF-dependent recycling of β1 integrin from intracellular compartment to the plasma membrane, cell spreading and FA formation were also suppressed by Grp1 knockdown ( Fig. 6f,g ). Consistent with these results, endogenous Grp1 co-localized with β1 integrin at the intracellular compartments ( Fig. 6h ). Thus, Grp1 seems to function as an Arf6 GEF to transduce HGF-induced β1 integrin recycling at the intracellular compartments, probably recycling endosomes, in endothelial cells. Knockdown of the remaining Arf6 GEFs ( Supplementary Fig. 14b ) inhibited HGF-stimulated β1 integrin recycling for GEP100, EFA6B and EFA6D, but not EFA6A and EFA6C, to the unstimulated levels, as assessed by immunostaining of cell surface β1 integrin ( Supplementary Fig. 14c ). This inhibition by knockdown of these Arf6 GEFs was also rescued by ectopic expression of these shRNA-resistant Arf6 GEFs ( Supplementary Fig. 14d ). Thus, taken together with the result in Fig. 6d , the β1 integrin recycling seems to be regulated by multiple Arf6 GEFs, Grp1, GEP100, EFA6B and EFA6D. Unlike Grp1, however, other three Arf6 GEFs co-localize with β1 integrin at the plasma membrane, not at the β1 integrin-positive intracellular compartment ( Supplementary Fig. 15 ), indicating that they have a different function(s) from Grp1 in the β1 integrin recycling process. Since protein recycling from endosomes to the plasma membrane involves multiple steps, for example, budding of vesicles from endosomes, transport of the vesicles to the plasma membrane and tethering/fusion of the vesicles to/with the plasma membrane, distinct localization of Arf6 GEFs suggests that different populations of Arf6 regulate successive steps in β1 integrin recycling through activation by distinct Arf6 GEFs. This proposal is supported by the report that Arf6 is implicated in several different steps for glucose transporter 4 recycling in differentiated 3T3-L1 cells [39] . Thus, it is plausible that Grp1 functions at an earlier step of β1 integrin recycling at the β1 integrin-positive intracellular compartment and other GEFs function at a later step(s) such as tethering/fusion of the vesicles to/with the plasma membrane. SecinH3 suppresses tumour angiogenesis and growth Finally, we examined whether pharmacological inhibition of Arf6 activation suppresses HGF-induced angiogenesis in vitro , and tumour growth and angiogenesis in vivo . SecinH3 treatment effectively blocked HGF-induced aortic microvessel extension ( Fig. 7a ), demonstrating that Grp1-Arf6 axis is critical in HGF-induced angiogenesis in this model system. Most relevantly, growth of B16 melanoma and LLC syngraft tumours and tumour angiogenesis were markedly suppressed by SecinH3 administration ( Fig. 7b–f and Supplementary Fig. 16a–c ). However, SecinH3 failed to inhibit α-SMA + and lumenized vessel formation ( Fig. 7g and Supplementary Fig. 16d ), although Arf6 ablation did inhibit them ( Fig. 2e,f ), leading us to speculate that the Arf6 GEF involved in the process of blood vessel maturation, for example, the recruitment of vascular smooth muscle cells, might differ from the one that mediates ingression of blood vessels into tumours. It is noteworthy that mice appeared healthy throughout the 16 days of SecinH3 administration, suggesting that SecinH3 does not have unacceptable short-term toxicity. These results, taken together, indicate that endothelial Grp1-Arf6 signalling should be considered to be a candidate target pathway for suppress tumour angiogenesis and growth, particularly in combination with other anti-angiogenic therapeutics that target VEGFR and/or PDGFR. 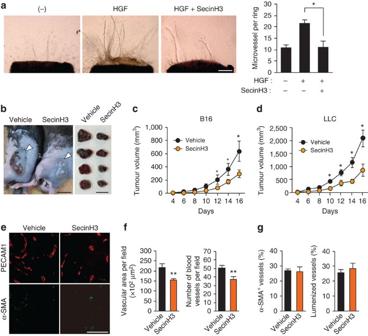Figure 7: SecinH3 inhibits tumour angiogenesis and growth. (a) Inhibition of HGF-induced microvessel sprouting from aortic ring explants by SecinH3. Aortic ring explants were prepared from wild-type mice. The data shown in the right panel represent means±s.e.m. from three independent experiments. Scale bar, 200 μm. (b–d) Tumour growth of B16 melanoma and LLC syngrafts in mice administered with vehicle or 1 mM SecinH3. Pictures of primary B16 melanoma tumours after 16 days of transplantation (b), and growth curves of B16 melanoma (c) and LLC tumours (d) are shown. The data shown inc,dare means±s.e.m from >6 experiments. Scale bars, 1 cm. (e–g) Tumour angiogenesis analysed by immunostaining for PECAM1 (e, upper panels) and α-SMA (e, lower panels) in sections of B16 melanoma tumours after 16 days of transplantation. The vascular area (f, left), number of vessels (f, right), vessels covered by α-SMA+mural cells (g, left) and percentage of lumenized vessels (g, right) were quantified. Means±s.e.m. were shown for all panels. Scale bar, 200 μm. *P<0.05, **P<0.01, one-way analysis of variance with Tukey’s multiple comparison test foraand Student’st-test forc,d,f. Figure 7: SecinH3 inhibits tumour angiogenesis and growth. ( a ) Inhibition of HGF-induced microvessel sprouting from aortic ring explants by SecinH3. Aortic ring explants were prepared from wild-type mice. The data shown in the right panel represent means±s.e.m. from three independent experiments. Scale bar, 200 μm. ( b – d ) Tumour growth of B16 melanoma and LLC syngrafts in mice administered with vehicle or 1 mM SecinH3. Pictures of primary B16 melanoma tumours after 16 days of transplantation ( b ), and growth curves of B16 melanoma ( c ) and LLC tumours ( d ) are shown. The data shown in c , d are means±s.e.m from >6 experiments. Scale bars, 1 cm. ( e – g ) Tumour angiogenesis analysed by immunostaining for PECAM1 ( e , upper panels) and α-SMA ( e , lower panels) in sections of B16 melanoma tumours after 16 days of transplantation. The vascular area ( f , left), number of vessels ( f , right), vessels covered by α-SMA + mural cells ( g , left) and percentage of lumenized vessels ( g , right) were quantified. Means±s.e.m. were shown for all panels. Scale bar, 200 μm. * P <0.05, ** P <0.01, one-way analysis of variance with Tukey’s multiple comparison test for a and Student’s t -test for c , d , f . Full size image Because mice in which Arf6 is conventionally deleted are embryonically lethal [22] , the more detailed pathophysiological functions of Arf6 at the whole animal level have not yet been reported. In this study, utilizing a conditional KO approach, we demonstrated that Arf6 expressed in vascular endothelial cells plays critical roles in tumour angiogenesis and growth through the regulation of HGF-induced endothelial β1 integrin recycling. In dissecting the pathways involved, we also delineated the functional steps for multiple Arf6 GEFs, Grp1, GEP100, EFA6B and EFA6D as regulating HGF-induced β1 integrin recycling ( Supplementary Fig. 17 ). Thus, this study provides evidence for molecular mechanisms underlying HGF-dependent tumour angiogenesis and growth. Our findings suggest that selective suppression of Arf6 signalling via Grp1, GEP100, EFA6B or EFA6D may counter angiogenic redundancy resistance acquired by tumours targeted with anti-VEGF approaches, therefore potentially increasing the efficacy of current therapeutics. Although the results obtained in this study demonstrate that Arf6 is a key player in HGF-dependent tumour angiogenesis, only mild phenotypes were observed in developmental angiogenesis. It has been reported that HGF/cMet signalling in endothelial cells is involved in tumour angiogenesis and growth [9] , [10] , [11] . In addition, it has been demonstrated that the mice lacking endothelial expression of the cMet-docking protein Gab1, which mediates HGF/cMet signalling, exhibit no apparent defects in developmental angiogenesis, but show impairment in postnatal angiogenesis after ischaemia [40] . These observations indicate that endothelial HGF/cMet signalling actively regulates pathological but not developmental angiogenesis. On the other hand, VEGF is essential for developmental angiogenesis: loss of a single VEGF allele results in severe defects in the vasculature, leading to embryonic lethality [41] , [42] . The different phenotype of VEGF KO mice with severe defect in the vasculature from that of our EC- Arf6 cKO mice with very mild defects in developmental angiogenesis is consistent with the proposal that Arf6 is indispensable for HGF-induced but not VEGF-induced angiogenesis. However, Arf6 in iECs was rapidly and transiently activated in response to VEGF stimulation ( Fig. 3f ), raising the question of what function VEGF-activated Arf6 does perform. Hashimoto et al. [26] have shown that knockdown of Arf6 in HUVECs increases their vascular permeability, which is generally controlled by vesicular trafficking of vascular endothelial-cadherin induced by VEGF stimulation. More recently, it has been demonstrated that interleukin 1β regulates endothelial cell permeability through Arf6 activation to allow inflammatory cells to be recruited to inflammatory sites [43] . Taken together, these reports suggest that VEGF-stimulated Arf6 pathways and functions might be revealed through the study of different model systems. We also demonstrated that HGF-dependent recycling of β1 integrin is completely suppressed by deletion of Arf6, resulting in inhibition of HGF-induced FA formation on collagen and fibronectin, but not on vitronectin. These finding are consistent with the well-established reports that integrin complexes containing β1 integrin, such as α1β1 and α2β1, are receptors for collagen, and others, such as α4β1, α5β1, α8β1 and αvβ1, are receptors for fibronectin. Among these, α1β1, α2β1 and α5β1 play roles in tumour angiogenesis [34] . Thus, it is reasonable to conclude that the inhibition of HGF-induced β1 recycling by Arf6 deletion suffices to explain our observed suppression of tumour angiogenesis. Inspection of tumour vessels in EC- Arf6 cKO mice revealed defects not only in the ingression of vasculature but also in vessel maturation. β1 Integrin plays a central role in vascular maturation: α2β1 and α5β1 integrin complexes are implicated in the lumenization process following the formation and fusion of intracellular vacuoles [45] . Other complexes with β1 integrin, α3β1 and α6β1, may also control vessel maturation by interacting with components in the basement membrane [45] . Based on these reports, it is plausible that the impairment of β1 integrin recycling to the plasma membrane is responsible for defects in vessel maturation in tumours. However, administration of SecinH3 into mice could not suppress the lumenization of intratumoral vessels, although SecinH3 completely inhibited the HGF-induced β1 integrin translocation to the plasma membrane. Thus, the defect in β1 integrin recycling in Arf6 −/− endothelial cells cannot completely explain impaired vessel maturation in EC- Arf6 cKO mice. PDGF-BB secreted from endothelial cells recruits mural cells such as vascular smooth muscle cells and pericytes to form mature vessels [45] . Since Arf6 regulates exocytosis in several type of secretion cells [46] , [47] , it would be of interest to analyse whether endothelial Arf6 regulates production and/or secretion of a vessel maturation-related protein(s) through an Arf6 GEF distinct from Grp1. A recent study demonstrated that Grp1 is crucial to regulate insulin-dependent glucose transporter 4 recycling to the plasma membrane through Arf6 activation in differentiated 3T3-L1 adipocytes [39] . However, we also showed that other Arf6 GEFs, GEP100, EFA6B and EFA6D, were involved in HGF-induced β1 integrin recycling ( Supplementary Fig 14 ), leading us to speculate that these Arf6 GEFs regulate different steps in the HGF-induced β1 integrin recycling pathway, such as budding from recycling endosomes, transport of budded vesicles to the plasma membrane and tethering/fusion of vesicles to/with the plasma membrane. Arf6 has been reported to function at each of these recycling steps, albeit functioning through distinct downstream effectors. The Arf6 GAP, ACAP1, which interacts with clathrin and β1 integrin at recycling compartment, is an effector of Arf6 coupled to clathrin-coated vesicle formation, which is the initial step of β1 integrin recycling [36] . Moreover, the GTP-bound active form of Arf6 interacts with Sec10, a subunit of the exocyst complex involved in vesicle targeting to and tethering with the plasma membrane [48] . In addition, the well-known Arf6 effector phosphatidylinositol 4-phosphate 5-kinase [18] , which produces the versatile signalling lipid phosphatidylinositol 4,5-bisphosphate, regulates tethering of vesicles containing β1 integrin to the plasma membrane and/or fusion with it at the leading edge of migrating cells through the interaction of generated phosphatidylinositol 4,5-bisphosphate with the exocyst protein Exo70 (ref. 49 ). From these reports, it is likely that different pools of Arf6 are sequentially activated by distinct Arf6 GEFs and regulate different effectors at each step of β1 integrin recycling. Thus, the single GTPase Arf6 may be able to drive the entire process of β1 integrin recycling. Considering the localization of GEP100, EFA6B and EFA6D at the plasma membrane, Arf6 activated by these GEFs may be involved in tethering and fusion of vesicles at the plasma membrane. Collectively, our study demonstrates that endothelial Arf6 plays an important role in HGF-induced tumour angiogenesis and growth. In addition to the importance of Arf6 in tumour angiogenesis, it has been reported that Arf6 activation in cancer cells is required for cancer invasion and metastasis [50] . Recent preclinical studies have suggested that anti-angiogenic therapy may promote cancer invasion and metastasis by inducing hypoxia of cancer cells, suggesting that effective cancer therapeutic approaches should involve both inhibition of tumour angiogenesis and cancer invasion/metastasis [51] , [52] . The critical roles of Arf6 in both tumour vascularization and cancer cell invasiveness/metastasis provide a new cancer therapeutic opportunity. Mice Arf6 flox/flox mice were generated in the C57BL/6 × CBA background. Genomic DNA covering the Arf6 gene of C57Bl/6J mice was isolated from RPCI-23 BAC clone (Invitrogen). Two lox P sites flanking exons 1 and 2 of Arf6 were introduced using standard restriction enzyme and PCR-based cloning techniques. A neomycin-resistance cassette ( neo ) flanked by FRT sites was also inserted between exon 2 and the second lox P site to prepare a targeting vector. The linearized targeting construct was electroporated into TT2 embryonic stem cells to obtain the recombinated Neo allele. Germline transmission of the Neo allele was confirmed by PCR and Southern blot analyses. Mice with floxed Arf6 allele were generated by mating mice with Neo allele with FLPe transgenic mice (a generous gift from Dr K. Araki, Kumamoto University). The sequences of the primers used for PCR genotyping were as indicated in Supplementary Table 1 . Arf6 flox/flox mice were backcrossed to C57BL/6 for >5 generations, and sex-matched 8- to 12-week-old mice were used for the in vivo experiments. All experiments with mice were conducted according to the Guidelines for Proper Conduct of Animal Experiments, Science Council of Japan, and protocols were approved by the Animal Care and Use Committee, University of Tsukuba. In situ hybridization In situ hybridization for Arf6 was performed as previously described [53] . Briefly, E13.5 embryos were fixed with 4% paraformaldehyde (PFA)/PBS, and embedded in optimal cutting temperature compound to prepare cryostat sections. After sections were prepared and fixed in 4% PFA/PBS at room temperature (RT) for 10 min, they were washed with PBS three times and immersed in 0.1 M triethanolamine containing 0.25% acetic anhydride for 10 min. They were washed again with PBS and blocked in the prehybridization solution (50% formamide, 5 × SSC, 1 × Denhardt’s, 250 μg ml −1 transfer RNA, 500 μg ml −1 herring sperm DNA) at 4 °C overnight. The cRNA probes were then hybridized in hybridization buffer (50% formamide, 300 mM NaCl, 20 mM Tris-HCl (pH 8.0), 5 mM EDTA, 10 mM Na 2 HPO 4 , 10% dextran sulfate, 1 × Denhardt’s, 500 μg ml −1 transfer RNA and 200 μg ml −1 herring sperm DNA) at 65 °C overnight. The sections were washed with 0.2 × SSC (3.3 mM NaCl and 3.3 mM sodium citrate, pH 7.5) at 65 °C for 30 min four times. After being rinsed with buffer A (0.1 M Tris-HCl (pH 7.5) and 0.15 M NaCl), the sections were blocked with 10% normal sheep serum in the buffer A at RT for 1 h and incubated with the alkaline phosphatase-conjugated anti-DIG antibody (1:1,000 dilution; 11 093 274 910, Roche) in the buffer A supplemented with 1% sheep serum at 4 °C overnight. They were then washed with the buffer A supplemented with 0.1% Triton X-100 three times and developed by incubating with NBT/BCIP (1:200 NBT/BCIP stock solution, Roche) in a buffer consisting of 0.1 M Tris-HCl (pH 9.5), 0.1 M NaCl and 50 mM MgCl 2 . Images were obtained with Biozero BZ-8000 microscope (Keyence). Whole-mount immunostaining Embryos were fixed with 4% PFA/PBS and washed with PBS containing 0.1% Tween-20, followed by dehydration and rehydration. After being blocked with 1% non-fat milk in PBS containing 0.1% Tween-20, embryos were stained by sequential incubation with anti-PECAM1 antibody (1:200 dilution; Mec13.3, BD Pharmingen), biotin-conjugated anti-rat immunoglobulin G antibody (1:200 dilution; BA-4001, Vector Laboratories) and horseradish peroxidase-conjugated streptavidin (1:200 dilution; PK-4000, Vector Laboratories). Retinal angiogenesis Retinal angiogenesis was analysed as previously reported [54] . Eyes enucleated from P5 mice ( n =6 for each genotype) were fixed in 4% PFA/PBS for 20 min, and then retinas were dissected. The obtained retinas were stained with anti-PECAM1 (1:200 dilution; Mec13.3, BD Pharmingen) and anti-Desmin antibodies (1:200; D33, Dako). Images were obtained using confocal microscope (TCS/SP5, Leica) equipped with a DFC 500 digital camera (Leica) and were processed with Leica application suite (Leica). Immunohistochemistry Cryostat sections of tumours and mouse embryos were incubated with anti-PECAM1 (1:200 dilution; Mec13.3, BD Pharmingen or 1:50 dilution; ab28364, Abcam), anti-α-SMA (1:200 dilution; ab5649, Abcam) or the conformation-specific anti-β1 integrin antibody 9EG7 (1:50 dilution; BD Pharmingen) at 4 °C overnight. After being washed with PBS containing 0.05% Tween-20, sections were stained with secondary antibodies. Assay of tumour growth and angiogenesis B16 melanoma (5 × 10 5 cells) or LLC cancer cells (2.5 × 10 5 cells) suspended in 100 μl of serum-free Dulbecco’s modified Eagle medium (DMEM; Nacalai Tesque) were subcutaneously transplanted into the dorsal flank of 8-week-old male mice. In the assay for the effects of the cytohesin inhibitor SecinH3 on tumour growth and angiogenesis, vehicle or 1 mM of SecinH3 (Merck) in 50% DMSO/50% glycerol solution was continuously administered to cancer cell-transplanted mice by mini-osmotic pumps (MODEL2001, ALZET) at the pumping rate of 1.0 μl h −1 up to 16 days. The mini-osmotic pump was exchanged by the pump with the fresh inhibitor every 4 days. Tumour volume was measured by digital caliper every other day, and was calculated using the following formula: tumour volume=length × width 2 × 0.52. After 14 or 16 days of transplantation, tumours were dissected, fixed with 4% PFA in PBS and subjected to immunohistochemical analysis of tumour angiogenesis. Bone marrow transplantation Recipient control or EC- Arf6 cKO mice were irradiated by X-ray (Hitachi Medical Corporation) at 450 cGy twice. Bone marrow cells were isolated from donor control or EC- Arf6 cKO mice, and 5 × 10 6 cells suspended in PBS were intravenously injected into irradiated recipient mice next day of irradiation. At 10 weeks after irradiation, tumour cells were transplanted. Aortic ring assay Thoracic aortas were cut into 1 mm sections and embedded in collagen type I gel (Nitta gelatin). Serum-free EBM-2 (Clonetics) with or without 50 ng ml −1 of VEGF-A 165 (Peprotech), bFGF (Peprotech) or HGF (a generously gift of Dr K. Miyazawa, University of Yamanashi) was added onto the collagen gel of each well. For cytohesin inhibition study, culture medium also included vehicle or 10 μM of SecinH3. Culture medium was exchanged every other day. Microvessel-like sprouting structure was observed under the phase contrast microscope at 7 days after culture, and the number of sprouts growing from each aortic ring was counted. Preparation of immortalized cells and cell culture Endothelial cells prepared from homozygotes with the floxed Arf6 allele were immortalized and maintained as previously described [55] . Briefly, cells prepared from whole body of E11.5 embryos were infected with a retrovirus containing polyoma middle T antigen to select iECs. Expression of mRNAs of PECAM1 , ICAM2 and endomucin , which are specific mRNAs for endothelial cells, was confirmed in the prepared iECs by reverse transcription (RT)–PCR. iECs thus established were suspended in DMEM supplemented with 10% FBS (Gibco), 2 mM glutamine, 1 mM non-essential amino acids, 1 mM Na-pyruvate, 50 μM 2-mercaptoethanol, 50 units per ml of penicillin, 50 μg ml −1 of streptomycin, 10 μg ml −1 of endothelial cell growth factor (Roche) and 50 μg ml −1 of heparin, and maintained on 0.1% gelatin-coated dishes. iECs in serum-free DMEM containing 8 μg ml −1 of polybrene were infected with recombinant adenoviruses encoding control LacZ and Cre recombinase for 4 h to prepare control and Arf6 −/− iECs, which were used for in vitro experiments. HUVECs were cultured in EBM-2 medium (Lonza) supplemented with EBM-2 bullet kit (Lonza) and used in the experiments for knockdown of Arf6 GEFs and immunocytochemistry. To knock down Arf6 GEFs, cells were infected with lentiviruses encoding shRNAs for Arf6 GEFs. Targeting sequences of each shRNA for Arf6 GEF were as indicated in Supplementary Table 2 . Assay of in vitro capillary tube formation Control and Arf6 −/− iECs in 2% FBS/DMEM cultured on 24-well plates coated with Growth Factor-Reduced Matrigel (BD Biosciences) at 1.5 × 10 5 cells per well were stimulated with 50 ng ml −1 of VEGF-A 165 , bFGF or HGF. After 8 h of the stimulation, capillary tube length was measured. In the assay with iECs ectopically expressed with β1 integrin, cells were infected with adenovirus encoding β1 integrin generated according to manufacturer’s procedure of Adenovirus Dual Expression Kit (Takara) and were cultured for 1 day before assay. Cell migration assay iECs suspended in 2% FBS/DMEM were seeded in the upper chamber of trans-well migration chambers (8 μm pore size; Coster). The lower chamber was filled with 2% FBS/DMEM supplemented with or without 50 ng ml −1 of HGF. After 12 h, membrane filters were fixed with 4% PFA in PBS and stained with DAPI. The number of iECs migrated onto the lower surface of the membrane filter were counted using the BZ-II Analyzer (Keyence). Assay for activation of Arf6 and Rac1 iECs pretreated with vehicle or 15 μM of SecinH3 at 37 °C for 30 min on 0.1% gelatin-coated dishes were stimulated with 50 ng ml −1 of HGF or of VEGF-A 165 for the indicated times. After cells were lysed, the GTP-bound active form of Arf6 in the lysate was pulled down with glutathione–Sepharose beads (GE Healthcare) conjugated with glutathione S -transferase-tagged leucine zipper region II (amino acids 398–455) of c-jun NH 2 -terminal kinase-associated leucine zipper protein, which specifically binds to the active form of Arf6 (ref. 56 ). Rac1 activation was assessed as previously described [57] . Detection of β1 integrin on the plasma membrane Cell surface β1 integrin levels were determined by biotin labelling or immunostaining method. In the assay with biotin, control and Arf6 −/− iECs cultured in 2% FBS/DMEM for 1 day on 0.1% gelatin-coated dishes were pretreated with vehicle or 15 μM SecinH3 for 30 min, and stimulated with 50 ng ml −1 of HGF or VEGF-A 165 in the presence of 20 μg ml −1 of cycloheximide, which blocks β1 integrin expression during stimulation, for the indicated times. Cell surface proteins were labelled with 0.5 mg ml −1 membrane-impermeable EZ-Link Sulfo-NHS-Biotin (Thermo Scientific) in PBS for 30 min on ice. To remove unbound biotin, 50 mM of NH 4 Cl was added to the cell culture, and cells were incubated for 10 min and washed three times with ice-cold PBS. After cells were lysed in lysis buffer composed of 50 mM Tris-HCl (pH 7.5), 150 mM NaCl, 1 mM EDTA, 0.1% sodium dodecylsulfate, 1% Triton X-100 and protease inhibitor cocktail (Nacalai Tesque), cell lysates were incubated with streptavidin beads (Thermo Scientific) for 6 h at 4 °C. The precipitates were thoroughly washed and proteins bound to beads were eluted. β1 Integrin eluted from beads were detected by western blotting probed with anti-β1 integrin antibody. In the immunostaining assay, control and Arf6 GEF-knocked-down HUVECs were starved for 8–12 h, and stimulated with 50 ng ml −1 of HGF for 5 min. In the rescue experiments for Arf6 GEFs, these cells were introduced with GFP or GFP-tagged shRNA-resistant Arf6 GEFs with Lipofectin Regent (Invitrogen) according to manufacturer’s procedure 1 day before HGF stimulation. After cells were fixed and blocked with 1% BSA/PBS without permeabilization step, cell surface β1 integrin was visualized with anti-β1 integrin antibody (1:50 dilution; TS2/16, Santa Cruz) and Alexa-350 or Alexa-488 conjugated secondary antibody (1:1,000 dilution; A11045 and A11029, respectively, Molecular Probes). To detect the transfected cells, cells were permeabilized with 1% BSA/PBS containing 0.1% Triton X-100 for 30 min, and subsequently stained with anti-GFP antibody (1:1,000 dilution; 598, Medical & Biological Laboratories Co.). Cell surface β1 integrin levels were assessed by determining the fluorescence intensity using ImageJ software. Assay for internalization of β1 integrin The internalization of β1 integrin was performed as previously reported with minor modification [58] . In brief, cells were starved for 1 h, labelled with biotin and incubated in serum-free DMEM with or without 50 ng ml −1 of HGF at 37 °C in the presence of 0.6 μM of primaquine, which inhibits protein recycling from endosomes to the plasma membrane, to allow the internalization of surface proteins. At the indicated times, biotin were removed from proteins remaining at the cell surface by incubating cells with the biotin-reducing compound MesNa (20 mM) in 50 mM Tris (pH 8.6) and 100 mM NaCl at 4 °C for 15 min. After MesNa was quenched by adding 20 mM iodoacetamide and followed by incubation for 10 min, cells were washed with PBS and lysed in the lysis buffer. β1 Integrin internalized was detected as described above. Assay of β1 integrin recycling β1 Integrin recycling was assessed by the decrease in internalized β1 integrin level resulted from its translocation from intracellular compartments to the plasma membrane. In the assay with iECs, β1 integrin inside the cell was detected by immunocytochemistry as previously reported [35] , [59] . In brief, iECs in cold PBS were incubated with an anti-β1 integrin antibody (1:200 dilution; HMβ1–1, BioLegend) for 30 min on ice. Surface-bound antibody was allowed to be internalized by incubating cells at 37 °C for 2 h in serum-free DMEM. After stimulation with 50 ng ml −1 of HGF for 5 min, cells were washed with cold PBS, and the antibody at cell surface was removed by washing cells with 0.2 M acetic acid/0.5 M NaCl in PBS on ice. In the assay with HUVECs, anti-human β1 integrin antibody (1:100 dilution; TS2/16, Santa Cruz) was used and 0.5% acetic acid/0.5 M NaCl/ PBS was used for washing surface antibody. Cells were then fixed, permeabilized and stained for β1 integrin inside the cell with secondary antibody (1:1,000 dilution; ab173003, Abcam for HMβ1-1 and 1:1,000 dilution; A11029, Molecular Probes for TS2/16). Assay for internalization and recycling of cMet Cells were pretreated with 10 nM of lactocystin and 100 nM of concanamycin to inhibit degradation of internalized cMet. After surface proteins of pretreated cells were labelled with biotin, internalization of cMet was determined according to the methods described above for ‘internalization of β1 integrin’ except for use of anti-cMet antibody for western blotting. In the assay for recycling of cMet, cells were labelled with biotin for surface proteins and incubated at 37 °C for 30 min to allow internalization of labelled surface proteins. After biotin was removed from proteins remaining at the cell surface with MesNa on ice, medium was changed to serum-free DMEM with 50 ng ml −1 of HGF, which was pre-warmed to 37 °C. At the indicated times, biotin was removed from proteins recycled to the plasma membrane by second MesNa treatment, and cells were lysed in 75 mM Tris-HCl (pH 7.5), 200 mM NaCl, 1.5% Triton X-100, 7.5 mM EDTA, 7.5 mM EGTA, 15 mM NaF, 1.5 mM Na 3 VO 4 and protease inhibitor cocktail. After biotinylated proteins inside the cell were recovered with streptavidin beads, cMet inside the cell was detected by western blotting probed with anti-cMet antibody, and recycling of cMet was calculated by the decrease in the amount of internal cMet. Immunocytochemistry To measure cell spreading and FA formation, control and Arf6 −/− iECs were treated with or without 50 ng ml −1 of HGF for 90 min, fixed with 2% formaldehyde/PBS on ice for 30 min, permeabilized with 0.1% Triton X-100 and 0.1% Tween-20, and blocked with 1% BSA/PBS for 1 h at RT. To assess the active form of β1 integrin on the plasma membrane using the antibody 9EG7, fixed iECs were subjected to blocking without a permeabilization step. To analyse subcellular localization of GFP-Arf6 GEFs and endogenous Grp1 and β1 integrin, HUVECs expressed with GFP-Arf6 GEFs were treated with HGF for 2.5 min, fixed and permeabilized as described above. These iECs and HUVECs were stained by sequential incubation with primary antibodies (1:1,000 dilution for anti-Paxillin antibody; 610051, BD Transduction Laboratories, 1:50 dilution for 9EG7; BD Pharmingen, 1:1,000 dilution for anti-GFP antibody; 598, Medical & Biological Laboratories Co., 1:200 dilution for anti-Grp1 antibody; HPA013979, Atlas Antibodies, 1:50 dilution for anti-β1 integrin antibody TS2/16; Santa Cruz, 20 μg ml −1 of anti-Arf6 antibody generated in our laboratory) and Alexa-488- or Alexa-546-conjugated secondary antibodies (1:1,000 dilution; Molecular Probes). F-actin was also visualized with rhodamine-conjugated phalloidin (1:1,000 dilution; Molecular Probes) in some experiments. iECs and HUVECs were then imaged using an Axiovert S100 Zeiss fluorescent microscope (Zeiss) equipped with an ORCA-ER CCD camera (Hamamatsu Photonics) and a confocal laser scanning microscope FLUOVIEW FV10i (Olympus), respectively. Fluorescent intensity of the active form of β1 integrin was measured using Lumina Vision software (Mitani Corporation). In the experiments for cell spreading and FA formation, cells were imaged using BZ-8000 microscope (Keyence) with a Plan Apo × 20 (numerical aperture 0.75; Nikon), and analysed for cell area and number of FA by BZ analyser imaging software (Keyence). HGF ELISA HGF protein levels in tumours and cancer cells were determined using mouse/rat HGF Quantikine ELISA Kit (R&D Systems) according to the manufacturer’s protocol. B16 melanoma and LLC tumours were dissected from mice after 18 days of transplantation of these cancer cells, homogenized in PBS and lysed with Cell Lysis Buffer 2 (R&D Systems). After centrifugation at 10,000 g for 10 min, supernatants were subjected to HGF enzyme-linked immunosorbent assay (ELISA). RT–PCR Total RNA was extracted using TRIzol regent (Gibco) and reverse transcription was performed by Superscript III (Invitrogen) according to manufacturer’s procedure. Sequences of PCR primers were listed in Supplementary Table 1 . Uncropped images of gels are shown in Supplementary Fig. 18 . Western blot analysis Sources of antibodies used for western blotting are as follows: anti-β1 integrin (1:500 dilution for clone18; BD Transduction Laboratories and 1:3,000 dilution for EP1041Y; Novus Biologicals), anti-phospho-ERK1/2 (1:250 dilution; E-4, Santa Cruz), anti-ERK2 (1:1,000 dilution; D-2, Santa Cruz), anti-phospho-JNK (1:1,000 dilution; no. 9251, Cell Signaling), anti-JNK (1:2,000 dilution; no. 9252, Cell Signaling), anti-phospho-p38 (1:1,000 dilution; no. 9211, Cell Signaling), anti-phospho-Akt (1:1,000 dilution; no. 9275, Cell Signaling), anti-Akt (1:1,000 dilution; no. 9272, Cell Signaling), anti-Rac1 (1:400 dilution; C-14, Santa Cruz), anti-phospho-cMet (Tyr1234/1235; 1:1000 dilution; no. 3126, Cell Signaling), anti-cMet (1:200 dilution; SP260, Santa Cruz). Rabbit polyclonal antibody specific to Arf6 was generated as previously described [52] . Western blotting was carried out as previously reported [59] . Uncropped images of blots are shown in Supplementary Fig. 18 . How to cite this article: Hongu, T. et al. Arf6 regulates tumour angiogenesis and growth through HGF-induced endothelial β1 integrin recycling. Nat. Commun. 6:7925 doi: 10.1038/ncomms8925 (2015).